Synthetic polyamines promote rapid lamellipodial growth by regulating actin dynamics Cellular protrusions involved in motile processes are driven by site-directed assembly of actin filaments in response to Rho-GTPase signalling. So far, only chemical compounds depolymerizing actin or stabilizing filaments, inhibiting N-WASP, Arp2/3 or formins, have been used to eliminate the formation of protrusions, while Rho-GTPase-dominant positive strategies have been designed to stimulate protrusions. Here we describe the design of four polyamines (macrocyclic and branched acyclic), and show that they enter the cell and induce specific growth of actin-enriched lamellipodia within minutes. The largest increase in cell area is obtained with micromolar amounts of a branched polyamine harbouring an 8-carbon chain. These polyamines specifically target actin both in vitro and in vivo . Analysis of their effects on filament assembly dynamics and its regulation indicates that the polyamines act by slowing down filament dynamics and by enhancing actin nucleation. These compounds provide new opportunities to study the actin cytoskeleton in motile and morphogenetic processes. Actin is involved in a variety of motile processes, including cell migration, cell division, wound healing, synaptic plasticity, immune response and host response to pathogens. The set of chemical agents available to characterize the role of actin dynamics in such processes is limited; latrunculin A and B are known to promote filament depolymerization by sequestering G-actin; cytochalasin D inhibits actin polymerization; and jasplakinolide stabilizes filaments and blocks assembly dynamics [1] . More recent drug screening experiments have identified chemicals specifically inhibiting the protein machineries that control initiation of filaments, such as wiskostatin, an inhibitor of N-WASP [2] , CK666, an inhibitor of Arp2/3 (ref. 3 ), and SMIFH2, an inhibitor of formins [4] . Alternatively, to stimulate actin assembly directly, thus avoiding pleiotropic effects of G-protein signalling, we have focused on polyamines, as macrocyclic polyamines (MPAs) have been shown to induce massive assembly of G-actin in large structures at low ionic strength, thus being coined ‘superpolyamines’ [5] . To extend these observations further, taking into account the structural characteristics of these MPAs, we have designed acyclic branched polyamines (BPAs) [6] intended to mimic the features of MPAs. They present a related pattern of two triamino subunits separated by a single polymethylene chain and are of much greater synthetic accessibility, being thus more suitable for the exploration of structural diversity. Polyamine compounds Four compounds with different structural features were designed and synthesized (see Methods and Fig. 1 ): a MPA, presenting two dipropylene triamine subunits linked by two aliphatic 7-carbon chains ( C 7 N 6 MPA ) ( Fig. 1a ); two BPAs containing two dipropylene triamine groups connected through the central nitrogen by a hexamethylene chain ( C 6 N 6 BPA ) ( Fig. 1b ) or a longer octamethylene chain ( C 8 N 6 BPA ) ( Fig. 1c ); and another BPA in which a chain of eight methylene groups connects two terminal subunits bearing additional branches ( C 8 N 14 BPA′ ) ( Fig. 1d ) to increase the density of amine groups. Additionally, a fluorescent derivative of C 8 N 6 BPA incorporating a Cy3 dye group C 6 N 6 BPA-Cy3 was synthesized to allow for optical detection ( Fig. 1e ). 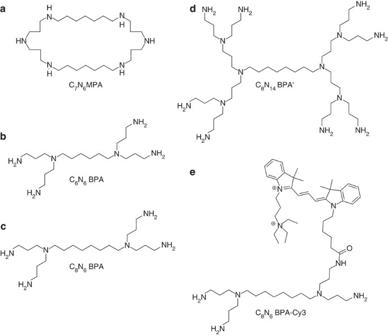Figure 1: Chemical structures of the synthetic polyamines. Five compounds were synthesized: (a) C7 MPA (C7N6MPA); (b) C6 BPA (C6N6BPA); (c) C8 BPA, first generation (C8N6BPA); (d) C8 BPA second generation (C8N14BPA′); and fluorescent compound (e)C8N6BPA-Cy3. Cx designates the length of the polymethylene chain(s) linking the triamino subunits. All compounds were stored and used as their hydrochloride salts (Supplementary Information). Figure 1: Chemical structures of the synthetic polyamines. Five compounds were synthesized: ( a ) C7 MPA ( C 7 N 6 MPA ); ( b ) C6 BPA ( C 6 N 6 BPA ); ( c ) C8 BPA, first generation ( C 8 N 6 BPA ); ( d ) C8 BPA second generation ( C 8 N 14 BPA′ ); and fluorescent compound ( e ) C 8 N 6 BPA-Cy3 . Cx designates the length of the polymethylene chain(s) linking the triamino subunits. All compounds were stored and used as their hydrochloride salts ( Supplementary Information ). Full size image Universal promotion of lamellipodial protrusions Addition of any one of the four compounds to the cell culture medium induced formation of flat protrusions with an unprecedented efficiency and speed. The effect was observed on four different cell types (see Fig. 2 and Supplementary Fig. S1 ). 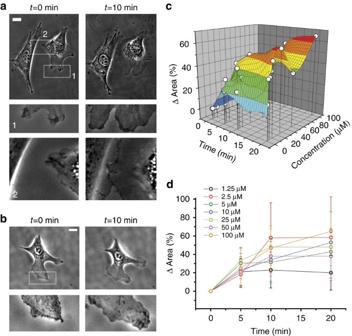Figure 2: Polyamine compounds promote growth of lamellipodia. Contrast-phase images of NIH3T3 cells before and after incubation with (a) 100 μM branchedC8N6BPA(Supplementary Movie 1) and (b) with 100 μMC7N6MPA(Supplementary Movie 2). Zooms of selected zones are represented below each panel. Note that lamellipodia extend preferentially on growth fronts, but lamellipodia also grow on the cells sides. Neighbouring cells establish contacts by bridging their lamellipodia (ina, region 2). Scale bars, 20 μm. (c) Live cell experiments were performed and the increase in the cell projected area was plotted for each compound and concentrations; here we show the three-dimensional plots forC8N6BPA. (d) Two-dimensional plot of the area increase as a function of time forC8N6BPA. (Number of cells analysed for each concentration:n(1.25 μM)=4;n(2.5 μM)=6;n(5 μM)=4 cells;n(10 μM)=10;n(25 μM)=14;n(50 μM)=16;n(100 μM)=9).N=4 for all conditions. Data are shown as mean±s.d. Figure 2 shows the responses of cells in the presence of branched C 8 N 6 BPA ( Fig. 2a ) and cyclic C 7 N 6 MPA ( Fig. 2b ) (see also Supplementary Movie 1 and 2 ). In both cases, within 10 min, protrusions were observed extending into sheets morphologically similar to classical lamellipodia. The effect was more pronounced on the edges of cells already exhibiting a lamellipodial activity before the addition of the drugs. However, ectopic lamellipodia were also observed to grow at other locations. As a secondary effect of cells spreading out, neighbouring cells were able to establish contacts de novo (see Fig. 2a , zoomed region). Figure 2: Polyamine compounds promote growth of lamellipodia. Contrast-phase images of NIH3T3 cells before and after incubation with ( a ) 100 μM branched C 8 N 6 BPA ( Supplementary Movie 1 ) and ( b ) with 100 μM C 7 N 6 MPA ( Supplementary Movie 2 ). Zooms of selected zones are represented below each panel. Note that lamellipodia extend preferentially on growth fronts, but lamellipodia also grow on the cells sides. Neighbouring cells establish contacts by bridging their lamellipodia (in a , region 2). Scale bars, 20 μm. ( c ) Live cell experiments were performed and the increase in the cell projected area was plotted for each compound and concentrations; here we show the three-dimensional plots for C 8 N 6 BPA . ( d ) Two-dimensional plot of the area increase as a function of time for C 8 N 6 BPA . (Number of cells analysed for each concentration: n (1.25 μM)=4; n (2.5 μM)=6; n (5 μM)=4 cells; n (10 μM)=10; n (25 μM)=14; n (50 μM)=16; n (100 μM)=9). N =4 for all conditions. Data are shown as mean±s.d. Full size image The efficiency of each compound in promoting the growth of lamellipodia was evaluated by measuring the increase in cell areas at several concentrations and different time intervals (see Methods). Optimal values for each circumstance were derived from the resulting three-dimensional graph ( Fig. 2c ) and the projected graphs ( Fig. 2d and Supplementary Fig. S2 ) for C 8 N 6 BPA . This way of quantifying the effect yields estimates for the efficiency. Note that lamellipodia growth can be modulated by nonlinear effects associated with fluctuations in protein concentrations or in feedbacks in signalling pathways. These measurements thus provide rough indications of the conditions for optimal effects rather than a detailed analysis of the concentration dependence of the effects of the drugs. As expected, the maximal increase was reached faster (within 5 min) at higher concentrations. The different compounds exhibited different behaviour in time response and in maximal increase in area ( Supplementary Fig. S2a–h ). These data suggest that both compounds C 8 N 6 BPA and C 7 N 6 MPA engender similar efficiencies for growth, but at lower concentrations for C 8 N 6 BPA . This also suggests that the distance set by the length of the chain between the two terminal triamino subunits, rather than the molecular topology, determines the efficiency of the drug. The following assays have been carried out with all compounds and similar results were obtained. For simplicity, only results obtained with C 8 N 6 BPA and C 7 N 6 MPA are shown below. Note that we used 100 μM concentration in most of the experiments in order to promote a dramatic and saturating effect for the growth of lamellipodia; however, lower concentrations such as 10 μM worked almost as well. To test the effect of polyamine ( C 7 N 6 MPA ) treatment on cell migration, control (untreated) and treated SW480 cells were seeded in a Boyden chamber with or without C 7 N 6 MPA 100 μM, and migration was assessed 24 h later (see Supplementary Methods ). As shown in Supplementary Fig. S3a , treatment with the actin-interacting agent could significantly inhibit the migration properties of SW480 cells compared with the control cells (32 +/− 2 cells per field versus 62 +/− 12 cells per field, Student’s t -test, P =0.03). We then evaluated if this effect was dependent on a reduced cell viability and analysed the SW480 cell survival fraction by trypan blue exclusion after 24 and 48 h exposure to increasing concentrations of superpolyamine. Our data clearly demonstrated that colon cancer cell line survival was not significantly modified even at the highest concentration (1 mM) ( Supplementary Fig. S3b ), suggesting that the effects of the polyamine on cell migration were not associated with cell death. Cell entry and growth promotion of lamellipodia Upon addition of the compounds, cell interaction with the extracellular matrix could be impaired, causing the formation of cell extensions that could differ from the canonical lamellipodia. To test this hypothesis, immunofluorescence localization of focal contact protein paxillin was performed on cells treated with C 8 N 6 BPA and C 7 N 6 MPA : cells exhibited the expected distribution and shapes of focal contacts [7] , which suggest that the drugs are promoting the growth of normal lamellipodia ( Fig. 3a–c ). 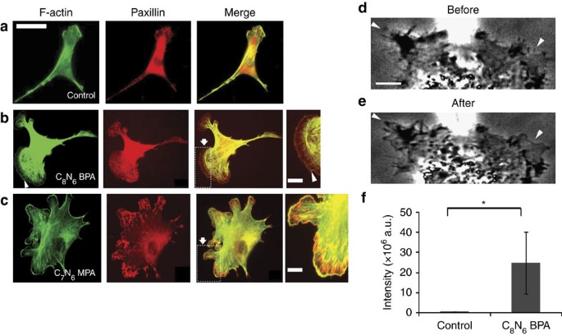Figure 3: Growth of lamellipodia is associated with the formation of focal contacts. (a) Control NIH3T3 cell stained for actin (green) and paxillin (red). Scale bar, 20 μm. (b) NIH3T3 cell 20 min after addition of 100 μMC8N6BPA. (c) NIH3T3 cell 20 min after addition of 100 μMC7N6MPA. White arrows in (b) and (c) show the lamellipodia protrusion after the addition of the polyamine compounds; arrowheads show also bundling of actin in (b). Highlighted regions are shown in more detail in the right panels. Scale bars, 10 μm. (d,e) Growth occurs upon injection. NIH3T3 cell before injection (d); and lamellipodia growth 10 s after injection of 300 μMC7N6MPA. Scale bar, 5 μm; (f) the compounds enter the cells. Experiments with 100 μMC8N6BPA-Cy3show that the polyamines enter the cells (n=10 cells,N=2). Data are shown as mean±s.d. *P<0.001 (Student’st-test). Figure 3: Growth of lamellipodia is associated with the formation of focal contacts. ( a ) Control NIH3T3 cell stained for actin (green) and paxillin (red). Scale bar, 20 μm. ( b ) NIH3T3 cell 20 min after addition of 100 μM C 8 N 6 BPA . ( c ) NIH3T3 cell 20 min after addition of 100 μM C 7 N 6 MPA . White arrows in ( b ) and ( c ) show the lamellipodia protrusion after the addition of the polyamine compounds; arrowheads show also bundling of actin in ( b ). Highlighted regions are shown in more detail in the right panels. Scale bars, 10 μm. ( d , e ) Growth occurs upon injection. NIH3T3 cell before injection ( d ); and lamellipodia growth 10 s after injection of 300 μM C 7 N 6 MPA . Scale bar, 5 μm; ( f ) the compounds enter the cells. Experiments with 100 μM C 8 N 6 BPA-Cy3 show that the polyamines enter the cells ( n =10 cells, N =2). Data are shown as mean±s.d. * P <0.001 (Student’s t -test). Full size image However, the pre-existence of cell focal contacts was not required for drug-promoted growth of cell extensions. Cells were gently detached and forced to round by incubation with a low concentration of trypsin ( Supplementary Fig. S4a–c ); after washing and addition of C 7 N 6 MPA , lamellipodia were promoted within 10 min, whereas control cells did not re-spread within this time period. This result demonstrates that the lamellipodium grows with de novo formation of focal contacts. The drugs could be acting on the actin cytoskeleton through an indirect mechanism, for instance by activating some upstream signalling molecule or by modifying the organization of the plasma membrane. Systematic checks were run to see that this was not the case. Repetition of the experiments in the absence of serum ( Supplementary Fig. S4d,e ) showed that within 10 min lamellipodia grew to the same extent as in the presence of serum. Further, injection of the compounds into the cells resulted in stimulation of lamellipodia in an identical manner, demonstrating that: (i) indirect effects on the membrane were not involved; (ii) the compounds entered the cell ( Fig. 3d,e ); and (iii) their effects simply resulted from their cytosolic localization. This last point was confirmed using 100 μM Cy3-labelled C 8 N 6 BPA (see Fig. 3f and Supplementary Fig. S5 ), which entered the cell and displayed the same effect as the unlabelled C 8 N 6 BPA . Taken together, these data suggest that the compounds penetrate the cells and promote growth of lamellipodia by targeting actin directly without the need for serum cofactors. Even though the uptake seems to be immediate, the compounds could be entering by passive diffusion or by carrier-mediated transport, as has been shown for polyamine and polyamine derivatives [8] , [9] . Strikingly, bundles of actin arranged in microspikes were observed within the lamellipodial array when C 8 N 6 BPA was added (see Fig. 3b , white arrow, right panel). This feature is consistent with earlier observations of actin networks in lamellipodia [10] . We therefore sought to prove the potential bundling of actin filaments by polyamines in vitro . Promotion of bundling of actin in vitro by polyamines MPAs have earlier been shown to induce assembly of actin into large aggregates in a low ionic strength buffer in which actin itself remains monomeric [5] . These aggregates were thought to be similar to those induced by polycations like spermine and spermidine [11] , [12] , [13] , poly- L -lysine, histones, polysaccharides and charged phospholipids; however, the MPAs appeared much more efficient in promoting actin aggregation than the large charged polyelectrolytes. The aggregates induced by cyclic polyamines were shown to be dissociated by ATP, which interacted with cyclic polyamines in competition with actin [5] . We checked that the compounds were not changing the pH in vitro in our weakly buffered solution, even at 300 μM. At physiological ionic strength (1 mM MgCl 2 , 0.1 M KCl), cyclic polyamines ( C 7 N 6 MPA ) as well as BPAs ( C 8 N 6 BPA ) induced assembly of actin ( Supplementary Methods ), although less efficiently than at low ionic strength. The assembly of G-actin in bundles of filaments was observed in a range of micromolar amounts of actin and 10–300 μM polyamines. It was characterized by the associated simultaneous increases in light scattering and in pyrenyl-actin fluorescence ( Fig. 4a,b ), and by electron-microscopy observation of negatively stained samples ( Fig. 4e,f ). Finally, we observed that ATP inhibited the formation of bundles in a dose-dependent manner ( Fig. 4c,d ). 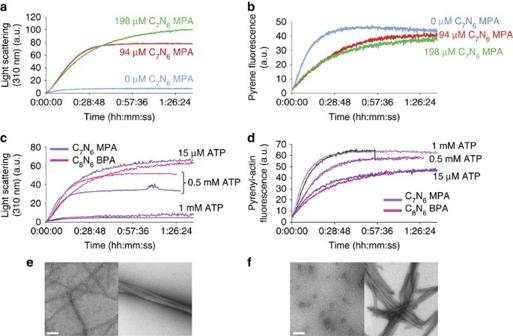Figure 4: Cyclic and BPAs induce ATP-sensitive bundling of actin filaments. (a–d) MgATP-G-actin (4 μM, 10% pyrenyl-labelled) was polymerized by addition of 1 mM MgCl2and 0.1 M KCl in the absence and presence ofC7N6MPA(a,b) or 150 μMC7N6MPAandC8N6BPA(c,d) at the indicated concentrations and in the presence of ATP at 0.2 mM (a,b) or at the indicated concentrations (c,d). Spontaneous polymerization was monitored by the increase in intensity of light scattering at 310 nm (a,b) and by the simultaneous increase in pyrenyl-actin fluorescence, recorded on the same samples (c,d). (e,f) Electron microscopy observation of solutions of actin (2 μM) in physiological ionic strength (e) or low ionic strength (f) in the absence (left panel) or in the presence (right panel) of 300 μMC7N6MPA. Scale bar, 100 nm. Figure 4: Cyclic and BPAs induce ATP-sensitive bundling of actin filaments. ( a–d ) MgATP-G-actin (4 μM, 10% pyrenyl-labelled) was polymerized by addition of 1 mM MgCl 2 and 0.1 M KCl in the absence and presence of C 7 N 6 MPA ( a,b ) or 150 μM C 7 N 6 MPA and C 8 N 6 BPA ( c,d ) at the indicated concentrations and in the presence of ATP at 0.2 mM ( a , b ) or at the indicated concentrations ( c,d ). Spontaneous polymerization was monitored by the increase in intensity of light scattering at 310 nm ( a , b ) and by the simultaneous increase in pyrenyl-actin fluorescence, recorded on the same samples ( c,d ). ( e , f ) Electron microscopy observation of solutions of actin (2 μM) in physiological ionic strength ( e ) or low ionic strength ( f ) in the absence (left panel) or in the presence (right panel) of 300 μM C 7 N 6 MPA . Scale bar, 100 nm. Full size image These results show that the bundling of actin occurs both in vitro and in vivo . We next probed the specificity of the compounds in vivo by using inhibitors. Lamellipodia growth without cell contractility When acto–myosin interaction was inhibited by blebbistatin or by ML-7, the lamellipodia were still growing after addition of the compounds ( Fig. 5a ). Growth was also observed when Rho kinase was inhibited by the classical Y27632 drug ( Fig. 5a bottom and Supplementary Movie 3 ). 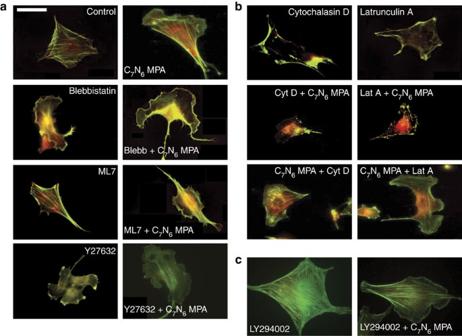Figure 5: (a)C7N6MPAandC8N6BPApromote lamellipodia growth even when contractility is inhibited. (From top to bottom) NIH3T3 fibroblast before and after incubation 20 min with 100 μMC7N6MPA; NIH3T3 cell after incubation 30 min with 30 μM Blebbistatin before and after 20 min with 100 μMC7N6MPA; cells incubated 30 min with 10 μM ML7 before and after 20 min with 100 μMC7N6MPA; cells incubated for 30 min with 10 μM Y27632 before and after 20 min with 100 μMC7N6MPA(Supplementary Movie 3). (b) Polyamines effect in the presence of Cytochalasin D and Latrunculin A. Actin specificity and barbed-end target. (From left to right and top to bottom) 1 μM Cytochalasin D, 1.5 μM Latrunculin A, 1 μM Cytochalasin D followed by 100 μMC7N6MPA, 1.5 μM Latrunculin A followed by 100 μMC7N6MPA, 100 μMC7N6MPAfollowed by 1 μM Cytochalasin D and 100 μMC7N6MPAfollowed by 1.5 μM Latrunculin A. (c)C7N6MPAeffect in the presence of PIK3 kinase inhibitor LY294002. (Left) NIH3T3 cell after incubation 50 min with 50 μM LY294002. (Right) Cells incubated for 50 min with 50 μM LY294002 before and after 20 min with 100 μMC7N6MPA. Scale bar, 20 μm. Figure 5: ( a ) C 7 N 6 MPA and C 8 N 6 BPA promote lamellipodia growth even when contractility is inhibited. (From top to bottom) NIH3T3 fibroblast before and after incubation 20 min with 100 μM C 7 N 6 MPA ; NIH3T3 cell after incubation 30 min with 30 μM Blebbistatin before and after 20 min with 100 μM C 7 N 6 MPA ; cells incubated 30 min with 10 μM ML7 before and after 20 min with 100 μM C 7 N 6 MPA ; cells incubated for 30 min with 10 μM Y27632 before and after 20 min with 100 μM C 7 N 6 MPA ( Supplementary Movie 3 ). ( b ) Polyamines effect in the presence of Cytochalasin D and Latrunculin A. Actin specificity and barbed-end target. (From left to right and top to bottom) 1 μM Cytochalasin D, 1.5 μM Latrunculin A, 1 μM Cytochalasin D followed by 100 μM C 7 N 6 MPA , 1.5 μM Latrunculin A followed by 100 μM C 7 N 6 MPA , 100 μM C 7 N 6 MPA followed by 1 μM Cytochalasin D and 100 μM C 7 N 6 MPA followed by 1.5 μM Latrunculin A. ( c ) C 7 N 6 MPA effect in the presence of PIK3 kinase inhibitor LY294002. (Left) NIH3T3 cell after incubation 50 min with 50 μM LY294002. (Right) Cells incubated for 50 min with 50 μM LY294002 before and after 20 min with 100 μM C 7 N 6 MPA . Scale bar, 20 μm. Full size image Inactivity of polyamine in the presence of actin inhibitors In contrast, the polyamine compounds had no effect when cellular actin polymerization was prevented by prior incubation with the depolymerizing drugs Cytochalasin D or Latrunculin A ( Fig. 5b ). This suggests that a key target is indeed actin and that the ability of actin to self-assemble is required for the drug to cause lamellipodia extension. We next examined the effect of the compounds on well-dispersed cells on surfaces coated with high density of fibronectin. Growth of lamellipodia was not recorded; when plated on densely coated surfaces, cells were extensively spread and showed large lamellipodia. This phenomenon was associated with extensive F-actin assembly by the cells, thus depleting the G-actin source available in standard conditions. Not surprisingly, the compounds did not promote further extension of the lamellipodia in this situation, probably because the cells were lacking a source of available G-actin. We further examined how the dynamics and stability of actin arrays pre-assembled by polyamines were affected by the depolymerizing drugs Cytochalasin D and Latrunculin A ( Fig. 5b ). While addition of Cytochalasin D (1 μM) to C 7 N 6 MPA -pretreated cells caused disruption of actin arrays, the lamellipodia induced by C 7 N 6 MPA remained assembled upon addition of Latrunculin A (1.5 μM). The failure of the lamellipodial actin arrays to disassemble upon addition of the actin sequestering drug suggests that these arrays are unusually stable. Consistently, when cells were permeabilized by Triton [1] , the lamellipodial arrays induced by polyamines resembled jasplakinolide-treated cytoskeletons ( Supplementary Fig. S6 ). We next studied the interaction between the compounds and acidic lipids. These compounds could bind lipids, thereby activating the PI3 kinase associated with lamellipodial growth. We observed that no growth was promoted when the PI3 kinase inhibitor (LY294002) [14] was added ( Fig. 5c ). However, we saw lamellipodial growth when our compounds were subsequently added. This confirms the direct effect of the compounds on actin. Positively charged molecules were shown to induce the bundling of cytoskeletal polymers by neutralizing charges. We therefore checked whether the compounds were altering the organization of microtubules and intermediate filaments: no difference was observed in their organization ( Supplementary Fig. S7 ). This further shows the specificity of these synthetic polyamines. Altogether, these results suggest that the in vivo effects of the polyamine drugs result from their functional interaction with regulated actin assembly leading to lamellipodial arrays. We therefore sought to characterize their effects on actin assembly dynamics in vitro using bulk solution assays and reconstituted motility assays. Specific retardation of barbed-end growth by polyamines Preliminary polymerization assays performed using either light scattering or pyrenyl-actin fluorescence as probes indicated that spontaneous assembly at physiological ionic strength is slowed down by polyamines ( Fig. 4b ). Whether polyamines inhibit nucleation or elongation of actin filaments cannot be discerned by the spontaneous assembly assay. Seeded filament growth assays therefore were performed using spectrin–actin seeds and gelsolin–actin complexes, which initiate barbed-end and pointed-end growth of filaments, respectively. 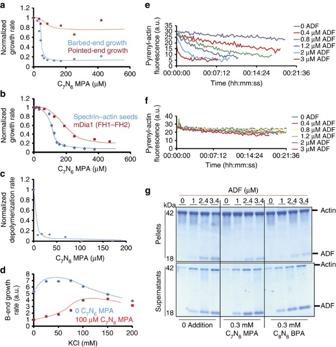Figure 6: Cyclic polyamines slow down filament dynamics at barbed ends specifically, without affecting the thermodynamic stability of the filaments. (a) Barbed-end and pointed-end growth were monitored using pyrenyl-actin fluorescence in the presence of 2.5 μM MgATP–G-actin. Rates are normalized taking as 1 the value measured in the absence ofC7N6MPA. (b) Binding of FH1–FH2formin construct to barbed ends protects from the inhibition byC7N6MPA. Conditions are as in (a). (c) Dilution-induced depolymerization at barbed ends was measured at the indicated concentrations ofC7N6MPA. (d) Increasing ionic strength weakens the inhibition of barbed-end growth byC7N6MPA>. Barbed-end growth rates were measured at the indicated concentrations of KCl in the absence (blue) and presence (red) of 100 μMC7N6MPA. (Right) The ADF-induced increase in rate of depolymerization is greatly weakened byC7N6MPAandC8N6BPA. (e,f) Time courses of ADF-induced rapid depolymerization of gelsolin-capped filaments in the absence (e) and presence (f) of 0.15 mMC8N6BPA. (g) SDS–PAGE analysis of the pellets and supernatants of samples of F-actin (3 μM) incubated with ADF and with or without 0.3 mMC7N6MPAorC8N6BPAfor 1 h before being centrifuged at 400 000gfor 20 min. The steady state of actin assembly is not affected. Figure 6a shows that barbed-end growth was specifically inhibited by about 85% by MPA in the range 0–150 μM. Pointed-end growth, in contrast, was only slightly decreased in the same concentration range. On the other hand, when barbed-end growth was initiated by the FH 1 –FH 2 construct of formin mDia1, the half-inhibition of barbed-end assembly by C 7 N 6 MPA required a threefold higher amount of cyclic polyamine ( Fig. 6b ), indicating that formin binding to barbed ends somehow protects them from the inhibition by polyamines. Dilution-induced depolymerization assays further showed that barbed-end depolymerization was slowed down to the same extent as barbed-end growth by C 7 N 6 MPA ( Fig. 6c ). Although the kinetics of barbed-end assembly and disassembly were dramatically slowed down by C 7 N 6 MPA , the critical concentration for filament assembly appeared unaffected in measurements of F-actin assembled at steady state ( Supplementary Fig. S8a ). Similar results were obtained with BPAs ( Supplementary Fig. S8b ). Figure 6: Cyclic polyamines slow down filament dynamics at barbed ends specifically, without affecting the thermodynamic stability of the filaments. ( a ) Barbed-end and pointed-end growth were monitored using pyrenyl-actin fluorescence in the presence of 2.5 μM MgATP–G-actin. Rates are normalized taking as 1 the value measured in the absence of C 7 N 6 MPA . ( b ) Binding of FH 1 –FH 2 formin construct to barbed ends protects from the inhibition by C 7 N 6 MPA . Conditions are as in ( a ). ( c ) Dilution-induced depolymerization at barbed ends was measured at the indicated concentrations of C 7 N 6 MPA . ( d ) Increasing ionic strength weakens the inhibition of barbed-end growth by C 7 N 6 MPA >. Barbed-end growth rates were measured at the indicated concentrations of KCl in the absence (blue) and presence (red) of 100 μM C 7 N 6 MPA . (Right) The ADF-induced increase in rate of depolymerization is greatly weakened by C 7 N 6 MPA and C 8 N 6 BPA . ( e , f ) Time courses of ADF-induced rapid depolymerization of gelsolin-capped filaments in the absence ( e ) and presence ( f ) of 0.15 mM C 8 N 6 BPA . ( g ) SDS–PAGE analysis of the pellets and supernatants of samples of F-actin (3 μM) incubated with ADF and with or without 0.3 mM C 7 N 6 MPA or C 8 N 6 BPA for 1 h before being centrifuged at 400 000 g for 20 min. The steady state of actin assembly is not affected. Full size image As we showed that bundling was promoted by the compounds, we evaluated whether bundling was responsible for the assembly kinetics. Bundling of filaments by polyamines is less prominent at physiological ionic strength than at low ionic strength, and shows a higher concentration dependence range than the range at which extension of lamellipodia and slower barbed-end kinetics are observed. Although the involvement of bundling in the kinetic effects of superpolyamines cannot be completely discarded, the fact that the thermodynamic stability (critical concentrations at barbed and pointed ends) of the actin arrays do not appear modified suggests that the effects differ from those observed with bundling agents that bind in a 1:1 molar ratio to actin along the sides of filaments and stabilize actin arrays, like Eps8 (ref. 15 ) or EF1alpha [16] . In conclusion, polyamines do not affect the stability of filaments but slow down their assembly–disassembly dynamics. The electrostatic nature of the effect of polyamines on barbed-end growth was demonstrated by performing seeded growth assays at various ionic strengths in the absence and presence of 100 μM C 7 N 6 MPA and in a polymerization buffer containing 1 mM MgCl 2 and increasing KCl in the range 0–200 mM. The percentage inhibition of barbed-end growth decreased upon increasing ionic strength and was undetectable above 150 mM KCl ( Fig. 6d ). Retardation of treadmilling by polyamines Actin-based motile processes result from site-directed initiation of actin assembly by two major signal-responsive protein machineries. WASP family proteins use the Arp2/3 complex to branch filaments at the membrane and assemble a dendritic protrusive meshwork, while formins initiate barbed-end processive assembly of actin bundles. In both cases, force is produced by barbed-end growth fuelled by regulated treadmilling. Treadmilling that drives the formation of dendritic actin arrays is enhanced by the synergistic effects of capping proteins, profilin and actin depolymerizing factor (ADF/cofilin). ADF is known to destabilize actin filaments, promoting a large increase in pointed-end depolymerization rate, the limiting step in filament treadmilling [17] . Figure 6e–g confirms that gelsolin-capped filaments depolymerize up to a maximum of 30-fold faster in the presence of ADF, in agreement with previous data [17] . The gelsolin-capped filaments are too short (1 μm in length) to be severed by ADF, as the average length of ADF-decorated filaments is 3 μm, only threefold shorter than the average length of standard actin filaments [18] , hence the measured effect is only owing to an increase in depolymerization rate constant. In the presence of cyclic or BPAs, the rate of depolymerization was much less enhanced by ADF (about threefold at 3 μM ADF, versus 30-fold in the control without polyamines). However, a sedimentation assay showed that ADF caused the same partial depolymerization and bound F-actin similarly in all samples with and without C 7 N 6 MPA or C 8 N 6 BPA ( Fig. 6g ). In other words, the steady state of actin assembly in the presence of ADF is practically unaffected by C 7 N 6 MPA or C 8 N 6 BPA . Finally, note that in our hands, other bundling factors like fascin did not affect the kinetics of F-actin depolymerization by ADF in vitro . In conclusion, in this assay again cyclic and BPAs slow down the dynamics of actin filaments and abolish the effect of ADF, but do not affect the thermodynamics of actin binding to ADF. Retardation of propulsion of N-WASP-coated beads In parallel to these assays, we examined the effect of C 8 N 6 BPA on the propulsive movement of N-WASP-coated beads in a reconstituted motility assay containing F-actin, Arp2/3, ADF, profilin and gelsolin [19] . Addition of 50 μM C 8 N 6 BPA a few minutes after initiation of comet tail formation caused a dramatic decrease in propulsion rate ( Fig. 7a ). 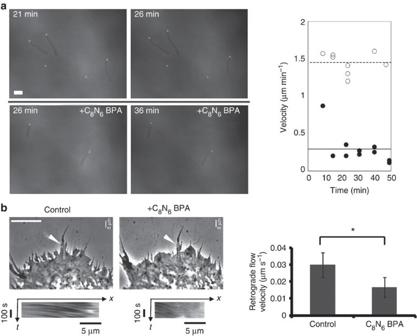Figure 7: (a) Polyamines slow down the propulsive actin-based movement of N-WASP-coated beads in a reconstituted motility assay. (Left) Time-lapse phase contrast images of actin-based movement of N-WASP-coated beads in a reconstituted motility assay (see Methods). Scale bar, 15 μm. (Right) Measured bead velocity of sustained actin-based propulsion in the absence (open circles) and in the presence (closed circles) of 50 μMC8N6BPAadded 2 min after placing the beads in the medium (time zero). (b) Actin retrograde flow is slowed down in the presence of polyamines. (Left) Contrast-phase images of the lamellopodia region of a REF 52 cell before and after the addition ofC8N6BPA. Scale bar, 5 μm. Kymographs of the highlighted region (dashed line) show a clear reduction in the actin retrograde flow. (Right) Graphic showing the measured retrograde flow velocity. (n=6 cells;N=6) Data are shown as mean±s.d. *P<0.05 (Students’st-test). Figure 7: ( a ) Polyamines slow down the propulsive actin-based movement of N-WASP-coated beads in a reconstituted motility assay. (Left) Time-lapse phase contrast images of actin-based movement of N-WASP-coated beads in a reconstituted motility assay (see Methods). Scale bar, 15 μm. (Right) Measured bead velocity of sustained actin-based propulsion in the absence (open circles) and in the presence (closed circles) of 50 μM C 8 N 6 BPA added 2 min after placing the beads in the medium (time zero). ( b ) Actin retrograde flow is slowed down in the presence of polyamines. (Left) Contrast-phase images of the lamellopodia region of a REF 52 cell before and after the addition of C 8 N 6 BPA . Scale bar, 5 μm. Kymographs of the highlighted region (dashed line) show a clear reduction in the actin retrograde flow. (Right) Graphic showing the measured retrograde flow velocity. ( n =6 cells; N =6) Data are shown as mean±s.d. * P <0.05 (Students’s t -test). Full size image We have shown that the polyamine compounds slow down the treadmilling of actin filaments in vitro . To verify that the turnover of lamellipodial actin arrays induced by the drugs is slowed down also in vivo , we complemented these experiments by measuring the retrograde flow ( Fig. 7b ) allowing proper visualization of the flow [20] (see Methods). Results showed that this flow is decreased in the presence of the polyamines. Altogether, these data show that in vivo as well, actin turnover is slower in the presence of the polyamine compounds. This leads to the stabilization of the lamellipodial-branched array. Promotion of enhanced actin nucleation in vitro While the above data explain why the lamellipodia were stabilized by the polyamines, in vitro data do not explain how lamellipodia could be initiated by the drugs. To address this point, we performed the following experiments. The lamellipodial-branched array requires the combined actions of filament branching directed at lamellipodium tip by WAVE protein using the Arp2/3 complex, and other regulators like ADF and capping proteins that enhance treadmilling. We had measured that the effect of ADF was weakened by polyamines. The effect of polyamines on capping protein activity was evaluated next. Capping proteins are required to maintain an environment in which most barbed ends are capped, thus establishing a high steady-state amount of G-actin, close to Cc of pointed ends. In addition, capping proteins block barbed-end growth of filaments nucleated by branching, thus regulating their length (architecture of the network) and lifetime. An optimum concentration range of capping protein is defined for maximum propulsion rate [21] , above which bead velocity decreases, because filament growth is arrested immediately after branching and nucleation of the daughter filament has occurred, thus generating a very densely branched and slowly growing network [19] . In solutions of pure actin, in the absence of capping proteins, critical concentration plots consist of two straight lines, indicating that a sharp transition exists at the critical concentration between the monomer and the polymer states. In contrast, barbed-end capping generates critical concentration plots that show a curvature in the region of the critical concentration, indicating that below and slightly above the extrapolated critical concentration short polymers are stabilized by the capping protein, as a result of the lowered free energy of nucleation. Most barbed-end cappers including Capping Protein and gelsolin actually nucleate actin. While in the absence of capping protein, the critical concentration plots obtained in the absence or presence of BPA are strictly superimposable, in the presence of capping protein they superimpose at high actin concentration but display a different curvature in the region of the critical concentration when BPA is present. The same effect was seen when we measured the dependence of the amount of F-actin at steady state on the concentration of added capping protein, at 1 μM total actin and in the presence of BPA/MPA ( Fig. 8 ). The data points are all above the ones observed in the control plot of data obtained in the absence of BPA, indicating that BPA stabilizes a greater number of short polymers in the presence of capping protein. 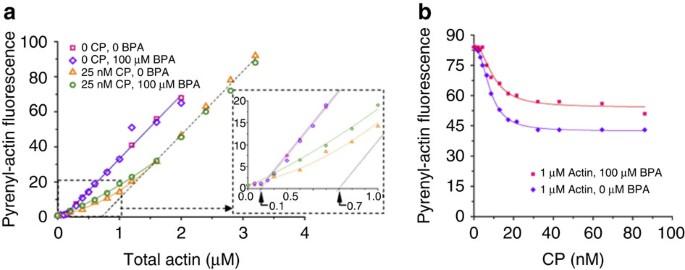Figure 8: Polyamines enhance nucleation by capping proteins. (a) Critical concentration plots with free barbed ends and in the presence of Capping Protein, with and withoutC8N6BPA. (b) Effect of Capping Protein on F-actin assembled at steady state (1 μM total actin) in the absence andpresence of 100 μMC8N6BPA. Note that the experimental data points show a sigmoidal dependence on CP concentration owing to the known nonlinear relationship between the critical concentration and the extent of barbed-end capping. Figure 8: Polyamines enhance nucleation by capping proteins. ( a ) Critical concentration plots with free barbed ends and in the presence of Capping Protein, with and without C 8 N 6 BPA . ( b ) Effect of Capping Protein on F-actin assembled at steady state (1 μM total actin) in the absence andpresence of 100 μM C 8 N 6 BPA . Note that the experimental data points show a sigmoidal dependence on CP concentration owing to the known nonlinear relationship between the critical concentration and the extent of barbed-end capping. Full size image The free energy of filament nucleation thus appears lowered to a larger extent with BPA than without BPA. The capping protein is in slow association–dissociation equilibrium with barbed ends. We propose that the fraction of oligomers that is not bound to capping protein at any time can therefore interact with a nucleating factor and become a stabilized growing filament. In other words, in the presence of capping protein, BPA would maintain a larger reservoir of potential actin filament pre-nuclei, thus facilitating filament branching by WAVE-Arp2/3. These results lead to the suggestion that polyamines enhance nucleation by capping protein, thus facilitating the initiation of filament branching at the lamellipodium tip. The present results bring mechanistic insight into two different aspects of actin-based motility. First, we provide evidence that small branched or cyclic polyamines promote growth of lamellipodia in various cell types; second, the effect of polyamines appears to be mediated by their regulation of actin nucleation and turnover in the cellular context, which sheds light on the potential mechanisms used by other cellular regulators of motility. These results offer the prospect of potential applications of polyamines as actin-specific tools in cell dynamics and medicine. We briefly review these perspectives below. Polyamines are cell-permeant and their effects in vivo reproduce the effects measured in vitro on simple systems composed of actin and regulators of treadmilling, such as ADF and Capping Protein. These small size polyamines act in two complementary ways: they slow down the turnover of actin within the existing lamellipodia and they enhance nucleation of actin at the cell edge. All polyamines like poly- L -lysine, protamines and histones are basic compounds, known to cause bundling of polyelectrolytes like actin filaments [22] , [23] by neutralizing negatively charged surface residues, for example, the exposed aspartate and glutamate residues of the N terminus of actin [24] . Small branched or cyclic polyamines (BPA/MPA) follow this rule and cause bundling of filaments in an ionic strength-sensitive fashion; however, they display additional peculiar properties that are responsible for their specific effects on actin dynamics. The data showing a high affinity inhibition of barbed-end assembly–disassembly kinetics suggest that binding of these polyamines to the terminal F-actin subunits alters the structure of the barbed end specifically. Further experimentation using microfluidics allied to TIRF microscopy to study individual filament dynamics, as well as more detailed structural molecular dynamics approaches, will be essential to evaluate this possibility. Consistent with this possibility is the narrow range of distances between active groups on polyamines in which the compounds display their regulatory activity on actin dynamics. Other amino compounds like neomycin have been reported to induce lamellipodia (for example, distribution of cytoskeletal proteins in neomycin-induced protrusions of human fibroblasts [25] ), most likely by acting on surface receptors. We have verified that up to at least 100 μM, neomycin does not induce bundling of actin at low ionic strength in vitro , while massive bundling is induced by BPA at that concentration, and does not inhibit barbed-end growth either ( Supplementary Fig. S9 ). Hence the effects of neomycin on cell motility are unlikely to be mediated by direct interaction with actin as those observed here with branched and cyclic superpolyamines. Remarkably, lamellipodia rather than filopodia appear to be induced by BPA/MPA. This observation, which is counterintuitive at face value, as filopodia are made of bundles and might be expected to be favoured by polyamines, is actually fully consistent with the in vitro observation that binding of formins (which promote filopodia) to barbed ends and successive assembly eliminate the effect of BPA/MPA on barbed-end dynamics ( Fig. 6a–d ). The slower assembly–disassembly dynamics of pure actin in vitro , and the resulting decreased velocity of N-WASP-coated beads propelled by site-directed assembly of a Arp2/3-branched actin meshwork may have implications in vivo [26] , [27] . In particular, we found that cell migration was slowed down in our assay with Boyden chambers. This is expected as motion is supported by barbed-end growth of WAVE-stimulated barbed-end assembly of an Arp2/3-branched actin array. Slower migration was actually measured in a variety of cell types following up to 24 h treatment by polyamines. It is possible, however, that slower migration results in part from the effect of polyamines on actin turnover at adhesions, which is coordinated to actin turnover in protrusive structures. Along the same line, polyamines may slow down other actin-based processes dependent on regulated treadmilling, such as re-organization of the Golgi apparatus [28] , scission of tubulated membranes by WASH/Arp2/3 (ref. 29 ), dendritic spine dynamics in synaptic plasticity [30] and the dynamics of immune synapse formed in T-cell activation [31] , [32] . BPA/MPA may have an instrumental role in the kinetic analysis of other processes, such as cytokinetic ring closure, in which ADF-mediated disassembly of actin filaments contributes to contractility [33] , [34] . Similarly, analysis of morphogenetic processes characterized by finely tuned rapid dynamics of actin filaments, such as the establishment of oocyte polarity in Drosophila [35] or spindle translocation in asymmetric meiotic division, may benefit from the use of BPA/MPA. Actually, in slowing down actin dynamics to desired levels, polyamines prove more manageable tools than Latrunculin A or Cytochalasin D to identify the key elementary steps. Polyamine targeting of the actin cytoskeleton represents an alternative to the use of specific reagents to block various cell functions. Polyamines are abundant in cells and have an important role in normal metabolism. Choosing those synthetic polyamines that have the appropriate size and geometry to target actin with high affinity will open avenues for manipulating cell motility and cell division and proliferation. This class of compounds will probably have a number of applications both in vitro and in vivo , with strong potential as a tool to study metastasis in cancer. In conclusion, we have shown that synthetic molecules, of both macrocyclic and acyclic BPA nature, can modulate actin dynamics in cells by implementing specific supramolecular interactions. These results extend the concept of ‘superpolyamines’ to both classes of compounds. The same approach could be used with other active groups of various geometries and distance between groups. Our work demonstrates that this approach can efficiently target proteins at the nanometre scale in vitro and in vivo. We anticipate and hope that this new class of compounds will be used in various situations both in vitro and in vivo . Chemical synthesis of the BPAs The BPAs were synthesized by a sequence involving: (1) treatment of terminal linear aliphatic diamines with acrylonitrile to give branched polynitriles, followed by (2) reduction of the nitrile groups to give the corresponding polyamines. The procedure for the preparation of branched polynitriles was the following [36] : acrylonitrile (5.0 equiv.) was added dropwise to the corresponding diamine (1.0 eq) dissolved in H 2 O at room temperature (RT). The resulted reaction mixture was warmed up to 50 °C and stirred for 3 h. The temperature was then increased to 80 °C and additional acrylonitrile (5.0 equiv.) was added dropwise. After 12 h, the reaction mixture was cooled to RT, the layers were separated and the aqueous layer was extracted with CH 2 Cl 2 (3 × 100 ml). The combined organic layers were dried over Na 2 SO 4 , filtered and concentrated in vacuo . The crude product was passed through a pad of silica (eluant: CH 2 Cl 2 /EtOAc) to give the corresponding nitriles as colourless oil. The procedure for the preparation of BPAs was the following: a given polynitrile (1.0 equiv.) was dissolved in a mixture of abs. EtOH and THF. Raney-nickel (8.2 equiv.) as a 50% suspension in water was added together with 2 N aqueous NaOH solution, and the reaction mixture was degassed and stirred under 1 atm of H 2 at RT for 24 h. The mixture was filtered off through a pad of celite, washed with EtOH (50 ml) and the solvents were removed in vacuo . The residue was dissolved in a mixture of water (50 ml) and CHCl 3 (100 ml), the layers were separated and the aqueous layer was extracted with CHCl 3 (4 × 100 ml). The combined organic layers were dried over Na 2 SO 4 , filtered and the solvent evaporated in vacuo . The polyamines were obtained as light yellow oils. Their hydrochloride salts were prepared as follows: to the amine (1 mmol) in hot methanol (10 ml) 6 M HCl (3 ml) and hot EtOH (10 ml) was added and the mixture was left at RT until a precipitate was formed. The precipitate was filtered off, washed with cold ethanol and dried in vacuo . The procedure for the preparation of Cy3 dye-labelled N,N,N′,N′-[tetrakis(aminopropyl)octamethylenediamine] C 8 N 6 BPA-Cy3 was the following: to a solution of Cy3 acid (30 mg, 0.05 mmol, 1 equiv.) and TSTU (O-(N-succinimidyl)-1,1,3,3-tetramethyluronium tetrafluoroborate, 24 mg, 008 mmol, 1.6 equiv.) in DMF (1 ml) triethylamine (7.0 μl, 0.05 mmol, 1 equiv.) was added. The mixture was stirred at RT for 1 h. The above mixture was added to a stirred solution of N,N,N′,N′-[tetrakis( aminop ropyl)octamethylenediamine] salt (59 mg, 0.1 mmol, 2 equiv.) and Na 2 CO 3 (106 mg, 1.0 mmol, 10 equiv.) in H 2 O (2 ml) and the reaction mixture was stirred for 15 h. The solvent was evaporated and the residue was purified by HPLC to obtain Cy3 dye-labelled C 8 N 6 BPA . The MPA C 7 N 6 MPA was obtained following the synthetic methodology previously described [37] . Cytoskeletal drugs Polyamine compounds were dissolved in Milli-Q water to give a stock solution of 30 mM. For immunostaining and microscopy experiments, polyamine compounds were added to the cell medium at a final concentration of 100 μM, except for experiments that tested efficiency. For immunostaining experiments, NIH3T3 cells were incubated with blebbistatin (30 μM), ML7 (10 μM), Y27632 (10 μM), cytochalasin D (1 μM) (Sigma-Aldrich) for 30 min, LY294002 (50 μM) (Sigma-Aldrich) for 30 min. Latrunculin A (1.5 μM) (Sigma-Aldrich) was added for 5 min. After additional 20 min incubation with 100 μM polyamine, cells were fixed and stained. Actin assembly–disassembly assays Actin assembly was monitored using as probes the increase in light scattering intensity (310 nm, 90° angle) and in the fluorescence of pyrenyl-actin (excitation 366 nm, emission 407 nm). Measurements were made at RT in a Xenius Safas spectrofluorimeter. CaATP–G-actin was converted into MgATP-G-actin by addition of 20 μM MgCl 2 and 0.2 mM EGTA to a solution of 10 μM CaATP–G-actin in G buffer. Polymerization was triggered by addition of MgCl 2 (1 mM final), EGTA (0.2 mM final) and KCl as indicated to MgATP-G-actin. The 1:1 CaATP–actin complex was obtained by removing free ATP by two consecutive treatments of CaATP–G-actin in G buffer with 10% suspension vol/vol of Dowex-I (BioRad) in G buffer without ATP. Seeded barbed-end growth assays were performed at 2.5 μM actin and 0.1 nM spectrin–actin seeds [38] . Pointed-end growth assays were performed similarly but using preformed gelsolin–actin complexes (2 nM final) as seeds. The initial rate of fluorescence increase was measured. Dilution-induced depolymerization assays were performed by 40-fold dilution of a 2.5 μM F-actin (50% pyrenyl-labelled) into F buffer containing BPA/MPA at desired concentrations. The initial rate of fluorescence decrease was measured. Critical concentration plots were performed by serial dilution of F-actin (10% pyrenyl-labelled) in F buffer containing the desired amounts of BPA/MPA. Pyrenyl-actin fluorescence was read after overnight incubation in the dark. Reconstituted motility assays Reconstituted motility assays were performed using 2-μm-diameter carboxylated polystyrene beads functionalized with N-WASP (170 nM, 2 h, followed by 1% BSA neutralization for 20 min) [19] . Beads were placed in a reconstituted motility mix containing 7.5 μM F-actin, 75 nM Capping Protein, 2 μM profilin, 7 μM ADF, 75 nM Arp2/3 complex in X buffer (10 mM HEPES, 0.1 M KCl, 1 mM MgCl 2 , 0.1 mM CaCl 2 , 1 mM ATP, 7 mM DTT, 1.5 mM DABCO at pH 7.8, 0.5% BSA and 0.2% methylcellulose). C 8 N 6 BPA was then added at 50 μM. Observations were made using a phase contrast Olympus AX70 microscope controlled by MetaMorph 6.3r7 with CCD camera and × 20 phase objective. Data analysis was performed to extract bead velocity with ImageJ software. Bead velocity was measured and averaged on 10–15 beads. Data analysis Increase in cell area for given time point ( n =5, 10 and 20 min) was calculated by ( A 1 n–A 0 )/A 0, where A 0 and A 1 n are the areas before and after polyamine addition, respectively. Kymographs for the analysis of actin retrograde flow in the lamellipodia region were performed in ImageJ. Moving features were visualized as diagonal streaks with slope depending on the velocity of movement. Statistical analysis Data are provided as mean±s.d. Statistical analysis was carried out by using two-tailed Student’s t -test, and significance was accepted at P <0.05. How to cite this article: Nedeva, I. et al. Synthetic polyamines promote rapid lamellipodial growth by regulating actin dynamics. Nat. Commun. 4:2165 doi: 10.1038/ncomms3165 (2013).